Hysteresis of ligand binding in CNGA2 ion channels Tetrameric cyclic nucleotide-gated (CNG) channels mediate receptor potentials in olfaction and vision. The channels are activated by the binding of cyclic nucleotides to a binding domain embedded in the C terminus of each subunit. Here using a fluorescent cGMP derivative (fcGMP), we show for homotetrameric CNGA2 channels that ligand unbinding is ~50 times faster at saturating than at subsaturating fcGMP. Analysis with complex Markovian models reveals two pathways for ligand unbinding; the partially liganded open channel unbinds its ligands from closed states only, whereas the fully liganded channel reaches a different open state from which it unbinds all four ligands rapidly. Consequently, the transition pathways for ligand binding and activation of a fully liganded CNGA2 channel differ from that of ligand unbinding and deactivation, resulting in pronounced hysteresis of the gating mechanism. This concentration-dependent gating mechanism allows the channels to respond to changes in the cyclic nucleotide concentration with different kinetics. Cyclic nucleotide-gated (CNG) ion channels mediate phototransduction in photoreceptors and chemotransduction in olfactory neurons [1] , [2] , [3] , [4] . Wild-type olfactory CNG channels are heterotetramers composed of two CNGA2 subunits, one CNGA4 subunit and one CNGB1b subunit [5] , [6] , of which only CNGA2 subunits can form functional homotetrameric channels. When studying steady-state concentration-activation relationships in inside-out membrane patches of CNGA2 channels, CNGA2 channels consistently produced Hill coefficients of ~2, indicating that at least two ligands are required for full channel activation [2] , [7] . Subsequent analysis of homotetrameric single CNGA2 channels confirmed that at least two ligands must bind for channel activation [8] . Using flash photolysis-induced cGMP jumps we later showed by a global fit strategy of activation time courses that at least three ligands are involved in channel activation and that the binding of the second ligand generates the main opening effect [9] . Combining such measurements with measurements of the ligand binding and the activation gating, we later demonstrated that all four ligands are involved in the activation gating, thereby confirming that the binding of ligand no. 2 is the key event for channel activation [10] . Moreover, our analysis revealed that models assuming ligand binding exclusively in the closed channel are sufficient to interpret the data. Therefore, the activation process seems to be operated by a complex cooperative mechanism: The binding of the first ligand hinders the binding of the second ligand, the binding of the second ligand promotes the binding of the third ligand, and the binding of the fourth ligand is not essentially influenced by the binding of the third ligand. With respect to the microscopic binding affinity, this results in a cooperativity sequence of ‘negative–positive–no’. A cooperativity sequence of comparable complexity has been identified for the ligand-induced activation of structurally related HCN2 channels pre-activated by voltage, although with different characteristics [11] , [12] , [13] . These results are inconsistent with the predictions of all types of models favouring a monotonous increase of the binding affinity with each ligand binding, including the Monod–Wyman–Changeux (MWC) model [14] , which is widely used to interpret the action of allosteric proteins, including the cooperative oxygen binding to haemoglobin [15] . Herein we used a fluorescence labelled cGMP (fcGMP) [10] , [16] in combination with confocal patch-clamp fluorometry [10] , [17] at elevated time resolution to further analyse ligand binding and activation gating in CNGA2 channels in terms of Markovian models. To determine not only equilibrium constants but also rate constants, we applied concentration jumps [12] and subjected multiple time courses of ligand binding and activation as well as ligand unbinding and deactivation to a global fit analysis. We show that, in comparison with the incompletely liganded or unliganded channel, the fully liganded channel reaches a different open state, which allows for a much faster successive unbinding of all four ligands, thereby giving rise to a pronounced hysteresis in the probability flow during gating. Time courses of ligand binding and channel gating We measured first the steady-state concentration-binding and concentration–activation relationship ( Fig. 1a ). As reported previously, these relationships cross each other and cannot be described with a simple Hill function [10] . Herein, these relationships were used to identify the three most promising concentrations to cover a wide concentration range for activation on the one hand and to provide time courses with reasonable resolution on the other. At low concentrations, the fluorescence signals are limited by the detector noise in the confocal images, whereas at high concentrations the limitations are set by the background fluorescence of the bath solution. For the kinetic studies the concentrations 0.5, 2.0 and 12.0 μM fcGMP were chosen ( Fig. 1a , grey arrows). 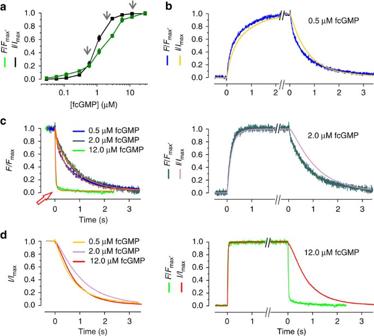Figure 1: Experimental data of fcGMP binding and gating in CNGA2 channels. (a) Concentration–binding relationship and concentration–activation relationship under steady-state conditions over a wide concentration range between 30 nM and 29.1 μM. Each data point is the mean of measurements obtained from 6 to 15 patches. Error bars denote s.e.m. The arrows indicate the concentrations used for the analyses of the time courses as shown inb. (b) Time courses of activation and deactivation as well as fcGMP binding and unbinding following a concentration pulse to either 0.5 μM (13.0 s), 2.0 μM (7.5 s), or 12.0 μM (9.0 s) fcGMP and back to zero. The traces are averages of 7, 7, 10 currents, respectively, arising from different patches. For better comparison the traces were graphically cut after reaching a steady state. All traces were normalized with respect to the late current (I/Imax) or late fluorescence intensity (F/Fmax). (c) Superimposition of the time courses of ligand unbinding. The colours correspond tob. The orange curves indicate monoexponential fits yielding the time constants for the ligand unbinding starting from different fcGMP concentrations. The red arrow indicates the unbinding time course at 12.0 μM fcGMP, which is ~50 times faster than the unbinding at the two lower concentrations. The obtained time constants are: 20.5 ms from 12 μM fcGMP, 943.2 ms from 2.0 μM fcGMP and 796.3 ms from 0.5 μM fcGMP. (d) Superimposition of the deactivation time courses. The colors correspond tob. Figure 1: Experimental data of fcGMP binding and gating in CNGA2 channels. ( a ) Concentration–binding relationship and concentration–activation relationship under steady-state conditions over a wide concentration range between 30 nM and 29.1 μM. Each data point is the mean of measurements obtained from 6 to 15 patches. Error bars denote s.e.m. The arrows indicate the concentrations used for the analyses of the time courses as shown in b . ( b ) Time courses of activation and deactivation as well as fcGMP binding and unbinding following a concentration pulse to either 0.5 μM (13.0 s), 2.0 μM (7.5 s), or 12.0 μM (9.0 s) fcGMP and back to zero. The traces are averages of 7, 7, 10 currents, respectively, arising from different patches. For better comparison the traces were graphically cut after reaching a steady state. All traces were normalized with respect to the late current ( I / I max ) or late fluorescence intensity ( F / F max ). ( c ) Superimposition of the time courses of ligand unbinding. The colours correspond to b . The orange curves indicate monoexponential fits yielding the time constants for the ligand unbinding starting from different fcGMP concentrations. The red arrow indicates the unbinding time course at 12.0 μM fcGMP, which is ~50 times faster than the unbinding at the two lower concentrations. The obtained time constants are: 20.5 ms from 12 μM fcGMP, 943.2 ms from 2.0 μM fcGMP and 796.3 ms from 0.5 μM fcGMP. ( d ) Superimposition of the deactivation time courses. The colors correspond to b . Full size image The averaged time courses of ligand binding and unbinding as well as activation and deactivation obtained with jumps to the chosen fcGMP concentrations and back to zero are shown in Fig. 1b . These averaged time courses represent the respective individual time courses well, as shown for the example of the fastest ligand binding and unbinding with 12 μM fcGMP in Supplementary Fig. S1 . Concerning ligand binding and activation gating, the results are the following: ligand binding is monotonously accelerated to the higher concentrations and the time course of activation closely follows the time course of ligand binding with an only short delay. Notably, none of the time courses for ligand binding and channel activation is sigmoid. This again rules out an independent gating of the subunits or a MWC-type mechanism [14] but confirms previous results obtained with cGMP, which led to the conclusion that the second binding step critically determines the activation gating [9] , [10] . Concerning ligand unbinding and deactivation, the situation proved to be more complex. In case of independent binding sites, one would expect that neither the ligand unbinding nor the deactivation gating depends on the ligand concentration. Our traces however showed that the unbinding at 12.0 μM fcGMP is ~50 times faster than the unbinding at the two lower concentrations ( Fig. 1c ). This is surprising because the unbinding at 2.0 μM fcGMP starts from 54% of the saturating signal ( c.f. Fig. 1a ) and this degree of binding should be passed when coming from a higher degree of ligand binding. A further remarkable result is that the time delay between ligand unbinding and deactivation is large at 12 μM fcGMP and much smaller at the lower concentrations ( Fig. 1b ). Superimposition of the deactivation time courses shows that they are only moderately different at the three fcGMP concentrations and that the time course at 2.0 μM fcGMP is slightly slower than those at 0.5 and 12.0 μM fcGMP ( Fig. 1d ). Though at the first glance these results are puzzling, they provide robust and stringent information that can be used to further unravel the molecular gating in CNGA2 channels. The C4L model is deficient to describe ligand unbinding The C4L model ( Fig. 2a ) was determined in our previous work by evaluating steady-state binding and activation with fcGMP as well as activation kinetics with cGMP [10] . Our analysis was therefore started by testing whether this model is also adequate to describe the time courses of ligand binding in addition to the time courses of activation and the two steady-state relationships and to view the predictions for the time courses of ligand unbinding and deactivation (for fitting strategy see Supplementary Methods ). Here and in all our fits we assumed equality of empty binding sites and equality of occupied binding sites, resulting in the stoichiometric factors 4, 3, 2, 1 and 1, 2, 3, 4 for the rates of binding and unbinding, respectively. 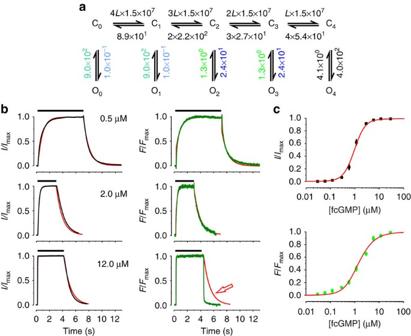Figure 2: Fit of ligand binding and activation with the C4L model. (a) Scheme of the C4L model. Cxand Ox(n=0…4) denote closed and open states, respectively.Lis a ligand. The numbers are the values of the rate constants (s−1or s−1M−1) determined by the fit. Rate constants set equal in the fit are indicated by using the same colours. The errors for each rate constant are given inSupplementary Table S1. (b) Time courses of binding and unbinding (green) as well as activation and deactivation (black) for three fcGMP concentrations. The time interval between the concentration jump from 0 to the respective fcGMP concentration and back to 0 is indicated for each trace by the black bar at the top. (c) Steady-state relationships for activation (black symbols) and ligand binding (green symbols). Each data point is the mean of measurements obtained from 6 to 15 patches. Error bars denote s.e.m. The red curves inbandcare the result of the best global fit of the time courses of ligand binding and activation as well as the steady-state relationships with the parameters shown ina. The reducedχr2for the activation/binding and steady-state was 5.0. Figure 2: Fit of ligand binding and activation with the C4L model. ( a ) Scheme of the C4L model. C x and O x ( n =0…4) denote closed and open states, respectively. L is a ligand. The numbers are the values of the rate constants (s −1 or s −1 M −1 ) determined by the fit. Rate constants set equal in the fit are indicated by using the same colours. The errors for each rate constant are given in Supplementary Table S1 . ( b ) Time courses of binding and unbinding (green) as well as activation and deactivation (black) for three fcGMP concentrations. The time interval between the concentration jump from 0 to the respective fcGMP concentration and back to 0 is indicated for each trace by the black bar at the top. ( c ) Steady-state relationships for activation (black symbols) and ligand binding (green symbols). Each data point is the mean of measurements obtained from 6 to 15 patches. Error bars denote s.e.m. The red curves in b and c are the result of the best global fit of the time courses of ligand binding and activation as well as the steady-state relationships with the parameters shown in a . The reduced χ r 2 for the activation/binding and steady-state was 5.0. Full size image The result was that the C4L model fitted the time courses of ligand binding and activation together with the steady-state relationships well ( Fig. 2b,c ). Our fit also verified that two ligands suffice to fully activate the channel [10] , as shown by values of the equilibrium constants for closed–open isomerizations ( E 0 , E 1 << E 2 , E 3 , E 4 , Fig. 2a and Supplementary Table S1 ). When considering the time courses of ligand unbinding and deactivation, which were not fitted in this approach, it becomes obvious that at 12 μM fcGMP the model does not match the fast ligand unbinding, whereas it approximately predicts the much slower deactivation time course ( Fig. 2b ). To test whether at 12 μM fcGMP the model is able to fit also the time courses of ligand unbinding and deactivation when optimizing the parameters, we included also these time courses in the fit ( Supplementary Fig. S2 ). The result was that the model still failed to describe the fast ligand unbinding and the slow channel deactivation at the same time. As this deficiency could not be overcome even when all rate constants were free parameters, the C4L model was classified as inadequate in its structure. The C4L-*O4L model The described inadequacies of the C4L model directed us to assume that pronounced ligand unbinding proceeds in the open channel. We therefore systematically extended the C4L model in several directions and fitted these models to the same data as used for the C4L model in Fig. 2 . These models are shown in Supplementary Fig. S3 . In a first approach, we enabled ligand unbinding also from open states by inserting respective transitions in the C4L model. Starting from the fully liganded state O 4 , we successively increased the number of transitions between the open states from one to four ( Supplementary Fig. S3 , models 1–4). The result was that model 2 and 4 provided the best result. When removing the saturating ligand concentration of 12 μM fcGMP these models led to a rapid decrease of ligand binding to 50% of the amplitude but could not adequately describe the deactivation kinetics (not shown). Insertion of only one or three transitions (models 1 and 3) compromized the fit (see χ r 2 ). We therefore suggested that other open states are passed during deactivation of the fully liganded and open channel than the ones populated during activation. To test this idea, we assumed that O 4 qualitatively differs from O 0 , O 1 , O 2 and O 3 by being the starting point for an additional pathway mediating the fast ligand unbinding at 12 μM fcGMP, whereas the following small slow phase of unbinding was thought to become fed by emptying O 3 and/or O 2 along the respective C pathway. The O states in the extra pathway are termed in the following *O 4 , *O 3 , *O 2 , *O 1 , *O 0 (C4L-*O4L model; Fig. 3a ). As the function of the *O-pathway was to enable a fast unbinding, we chose as simple approach to equalize both all forward rate constants and all backward rate constants. The result was a significant improvement of the fit compared with the C4L model ( Fig. 3b,c ). It should be noted that the binding constants along the *O-pathway were set to 6 × 10 8 M −1 s −1 , a reasonable value for a diffusion-limited binding [18] . As k C0*O0 is very slow it could be suggested that activation to *O 4 proceeds exclusively along the C pathway, whereas deactivation from *O 4 proceeds to a significant degree along the *O-pathway. Moreover, inclusion of the unbinding and deactivation time courses allowed us to differentiate between K AC1 , K AC3 , and K AC4 , which could not be achieved in our previous study [10] . The values of the equilibrium association rate constants were K AC1 =1.6 × 10 5 , K AC2 =8.2 × 10 4 , K AC3 =2.4 × 10 5 , and K AC4 =5.1 × 10 5 . Before discussing the processes in the C4L-*O4L model in greater detail, it should be noted that multiple other models with an *O-pathway were considered that were however inferior to the C4L-*O4L model with respect to a minimum in complexity and number of parameters as well as to a maximum in the parameters’ determinateness. A selection of models is shown in Supplementary Fig. S3 , including models with ligand unbinding via C x and *O x starting from incompletely liganded states O x and running to C 0 (model 5 and 6), models with ligand unbinding via C x , O x and *O x running to C 0 (model 7 and 8), models with ligand unbinding via C x and *O x starting from more than one O x and running to C 0 (models 9–11), and models with ligand unbinding via C x and *O x running to O 0 (models 12–14). 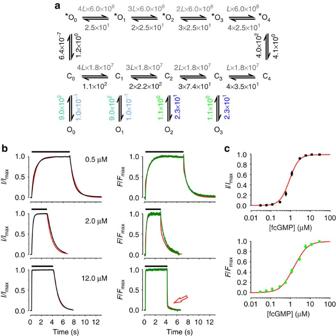Figure 3: Fit with the C4L-*O4L model including ligand unbinding and deactivation. (a) Scheme of the C4L-*O4L model. Cxand Ox(n=0…4) denote closed and open states, respectively. *Oxdenotes states of an extra pathway used only in deactivation.Lis a ligand. Again, the numbers provide the values of the rate constants (s−1or s−1M−1) determined by the fit. Rate constants set equal in the fit are indicated by using the same colours. The errors for each rate constant are given inSupplementary Table S2. (b) The time courses of ligand binding and unbinding as well as activation and deactivation are the same as those inFig. 2b. (c) The steady-state relationships are the same as those inFig. 2c. Each data point is the mean of measurements obtained from 6 to 15 patches. Error bars denote s.e.m. The red curves inbandcare the result of the best global fit with the C4L-*O4L model. The reducedχr2was 6.0. Figure 3: Fit with the C4L-*O4L model including ligand unbinding and deactivation. ( a ) Scheme of the C4L-*O4L model. C x and O x ( n =0…4) denote closed and open states, respectively. *O x denotes states of an extra pathway used only in deactivation. L is a ligand. Again, the numbers provide the values of the rate constants (s −1 or s −1 M −1 ) determined by the fit. Rate constants set equal in the fit are indicated by using the same colours. The errors for each rate constant are given in Supplementary Table S2 . ( b ) The time courses of ligand binding and unbinding as well as activation and deactivation are the same as those in Fig. 2b . ( c ) The steady-state relationships are the same as those in Fig. 2c . Each data point is the mean of measurements obtained from 6 to 15 patches. Error bars denote s.e.m. The red curves in b and c are the result of the best global fit with the C4L-*O4L model. The reduced χ r 2 was 6.0. Full size image Time-dependent population of states in the C4L-*O4L model Using the rate constants determined for the C4L-*O4L model ( Fig. 3a ; Supplementary Table S2 ) the probabilities of being in the individual open states (P O,x , P *O,x ; Fig. 4a ) and closed states (P C,x ; Fig. 4b ) as well as the contributions of each state to the total ligand binding were computed as function of time ( Fig. 4c ). 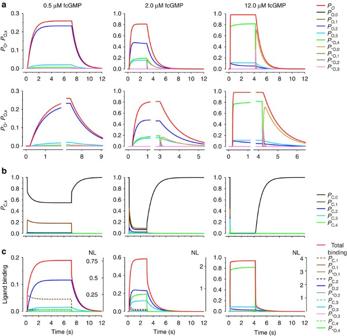Figure 4: Time-dependent state population in the C4L-*O4L model. Using the parameters given inFig. 3a, the population of all states in the C4L-*O4L model was computed for three fcGMP concentrations. (a) Upper time courses: open probability,Po(red curve, same curves as inFig. 3b) and probability of being either in Ox,PO,x(x=0….3) or *Ox, P*O,x(x=0….4; coloured curves). ThePO,xandP*O,xvalues sum up toPo. Lower time courses: part of the respective upper time courses at an expanded timescale. (b) Probability of being in the closed statex,PC,x(x=0….4). ThePO,x,P*O,x, andPC,x, values sum up to unity. (c) Ligand binding to the total channel (red curve) to the individual open (x/4 ×PO,x;x/4 ×P*O,x; coloured continuous) and closed states (x/4 ×PC,x; coloured dashed), given as fraction of unity (left ordinates).x/4 weighs the contribution of each liganded state to the total liganding. NL indicates the number of ligands bound to the channel and to the individual states under the assumption that maximally four ligands can bind to the channel (right ordinate). Figure 4: Time-dependent state population in the C4L-*O4L model. Using the parameters given in Fig. 3a , the population of all states in the C4L-*O4L model was computed for three fcGMP concentrations. ( a ) Upper time courses: open probability, Po (red curve, same curves as in Fig. 3b ) and probability of being either in O x , P O,x ( x =0….3) or *O x , P *O,x ( x =0….4; coloured curves). The P O,x and P *O,x values sum up to Po . Lower time courses: part of the respective upper time courses at an expanded timescale. ( b ) Probability of being in the closed state x , P C,x ( x =0….4). The P O,x , P *O,x , and P C,x , values sum up to unity. ( c ) Ligand binding to the total channel (red curve) to the individual open ( x /4 × P O,x ; x /4 × P *O,x ; coloured continuous) and closed states (x/4 × P C,x ; coloured dashed), given as fraction of unity (left ordinates). x /4 weighs the contribution of each liganded state to the total liganding. NL indicates the number of ligands bound to the channel and to the individual states under the assumption that maximally four ligands can bind to the channel (right ordinate). Full size image When stepping to 12.0 μM fcGMP ( Fig. 4 , right), the rapid increase of Po is caused by the population of three states: P *O,4 is populated by a dominating initial fast phase followed by a slow phase to reach finally 0.8 ( Fig. 4a , right). A minor portion of Po is generated by P O,3 and P O,2 . Hence, even at the saturating concentration of 12.0 μM fcGMP P O,3 and P O,2 are significantly populated. The time courses of binding mirror this respectively ( Fig. 4c , right). For the closed states the situation is simple, they are emptied rapidly ( Fig. 4b , right). When removing fcGMP, there are two pathways of deactivation. *O 4 is emptied exclusively and with high speed along *O 3 →*O 2 →*O 1 →*O 0 . *O 0 is relatively stable and only the transition *O 0 →C 0 causes slow deactivation ( Fig. 4a,b , right). In contrast, O 3 empties via C 3 →C 2 →C 1 to C 0 , thereby dominating the small slow phase of unbinding. Similarly, O 2 empties via C 2 →C 1 to C 0 . However, its contribution to the total unbinding is only minor. Hence, after removing the saturating fcGMP concentration of 12 μM, there are two relevant but distinct pathways for both unbinding and deactivation. At the intermediate fcGMP concentration of 2.0 μM fcGMP, the occupancy of *O 4 reaches only <0.2, whereas O 3 and O 2 sum up to >0.6 ( Fig. 4a , middle). As the latter can only deactivate along C 3 →C 2 →C 1 →C 0 and C 2 →C 1 →C 0 , respectively, unbinding is dominated by this slow process ( Fig. 4c , middle). Concerning the closed states, C 1 and C 0 remain populated in the presence of the ligand in total occupancy 0.2, whereas the other closed states are not essentially populated ( Fig. 4b , middle). Nearly all ligand binding comes from the open states O 2 , O 3 and *O 4 ( Fig. 4c , middle). In the logic of the previous, the total time course of unbinding is dominated by emptying O 3 and O 2 ( Fig. 4c , middle), whereas for total deactivation also the reaction *O 0 →C 0 is of relevance ( Fig. 4a , middle). At the low fcGMP concentration of 0.5 μM, there is only a moderate opening by populating O 2 ( Fig. 4a , left). The other open states do not play an essential role. Accordingly, also deactivation and ligand unbinding are dominated by emptying O 2 ( Fig. 4a,c , left). In the presence of the ligand, the closed states C 0 and C 1 are populated by ~55% and ~20%, respectively ( Fig. 4b , left). As *O 4 is not populated at this concentration, unbinding and deactivation along *O-pathway does not proceed. Hence, at this low concentration there is only one relevant pathway for deactivation, O 2 →C 2 →C 1 →C 0 . The C4L-*O4L model can indeed explain the surprising result of a 50 times faster ligand unbinding at saturating compared to non-saturating fcGMP by introducing an additional open state, *O, that can be reached only when all four binding sites are occupied and is emptied quickly when removing the ligand. Nevertheless, it remains remarkable that there is such a big kinetic difference between the two concentrations 2 and 12 μM fcGMP. To further approve the validity of our C4L-*O4L model, we first simulated time courses of ligand unbinding to identify a reasonably intermediate time course between 2 and 12 μM fcGMP and then tested whether the prediction is met by the experiment ( Fig. 5 ). We chose 4.5 μM fcGMP. The predicted time course of unbinding shows an initial rapid phase, due to the unbinding along the *O-pathway, followed by a slow phase with an amplitude between that at 12 and 2 μM fcGMP, evoked by the unbinding from O 3 and O 2 , (blue curve in Fig. 5 ). As these basic features are indeed met by the experiment (green trace in Fig. 5 ) with an only slight deviation, our C4L-*O4L model is considered to be adequate. 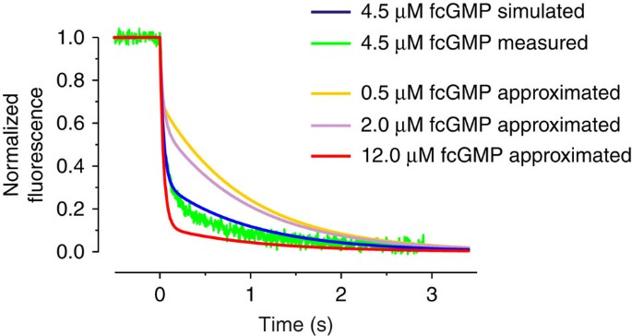Figure 5: Predicted and measured time course of ligand unbinding at 4.5 μM fcGMP. The approximated time courses of ligand unbinding at 0.5 μM, 2.0 μM, 4.5 μM and 12 μM fcGMP are obtained by the global fit with the C4L-*O4L model (c.f.Fig. 3). The time course at 4.5 μM (blue curve), simulated with C4L-*O4L model, approximately matches the experimentally determined time course at this concentration (green trace). The experimentally determined time course is the average from five individual time courses. Figure 5: Predicted and measured time course of ligand unbinding at 4.5 μM fcGMP. The approximated time courses of ligand unbinding at 0.5 μM, 2.0 μM, 4.5 μM and 12 μM fcGMP are obtained by the global fit with the C4L-*O4L model ( c.f. Fig. 3 ). The time course at 4.5 μM (blue curve), simulated with C4L-*O4L model, approximately matches the experimentally determined time course at this concentration (green trace). The experimentally determined time course is the average from five individual time courses. Full size image Transition pathways in the C4L-*O4L model In order to visualize the qualitative differences in the gating at the saturating fcGMP concentration of 12 μM and the low fcGMP concentration of 0.5 μM, we considered the probability fluxes [11] in our C4L-*O4L model. Knowledge of the occupancy of each state at each time allowed us to compute for all individual transitions between two neighboured states X↔Y the total net probability flux, F XY , that is, the net amount of probability moving between the two states either when fcGMP was applied or when it was removed ( Supplementary Methods ). Knowing all total net probability fluxes in our C4L-*O4L model, we computed the pathway net probability flux, F p,XY , between two arbitrary, not necessarily neighboured, states X and Y within the model (equation S10 in Supplementary Methods ). As in the absence of fcGMP the channel is nearly completely in C 0 and at 12 μM fcGMP nearly completely in O 2 , O 3 , or *O 4 ( Fig. 4a,b , right), for channel activation the pathway net probability fluxes F p,C0O2 , F p,C0O3 and F p,C0*O4 were considered (red arrows in Fig. 6 ). In this context, C 0 is the flux producer and O 2 , O 3 , *O 4 are the flux collectors. It is evident that at 12 μM fcGMP F p,C0*O4 dominates channel activation by far ( Fig. 6a ), whereas it becomes irrelevant at 0.5 μM fcGMP, where the fractional activation is generated by F p,C0O2 and F p,C0O3 ( Fig. 6c ). At 2.0 μM fcGMP, F p,C0O2 is already larger and F p,C0O3 in the same order as F p,C0*O4 ( Fig. 6b ). 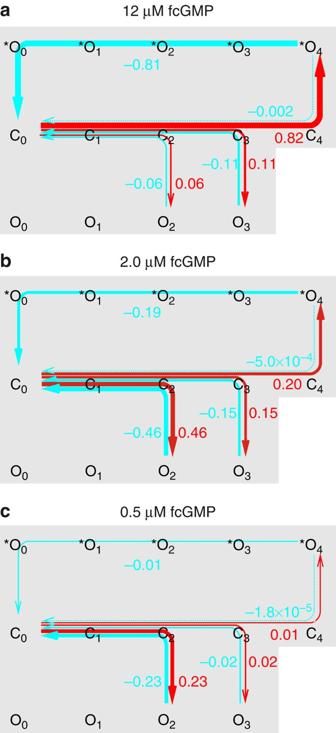Figure 6: Transition pathways in the C4L-*O4L model. The net probability fluxes along specified transition pathways between state X and Y,Fp,XY, were computed by integrating the net probability flux densities and employing the principles of the transition pathway theory (seeSupplementary Methods). The weight of the pathway net probability fluxes is semiquantitatively encoded by the thickness of the arrows (fluxes below 2 × 10−4are indicated by dotted lines. The numbers besides the coloured graphs indicate the exact weights as fraction of unity. (a) 12 μM fcGMP. Pathway net probability fluxes along the pathways C0…*O4, C0…O3, and C0…O2after applying fcGMP (red) and after its removal (blue). (b,c) Respective pathway net probability fluxes at 2.0 μM and 0.5 μM fcGMP, respectively. Figure 6: Transition pathways in the C4L-*O4L model. The net probability fluxes along specified transition pathways between state X and Y, F p,XY , were computed by integrating the net probability flux densities and employing the principles of the transition pathway theory (see Supplementary Methods ). The weight of the pathway net probability fluxes is semiquantitatively encoded by the thickness of the arrows (fluxes below 2 × 10 −4 are indicated by dotted lines. The numbers besides the coloured graphs indicate the exact weights as fraction of unity. ( a ) 12 μM fcGMP. Pathway net probability fluxes along the pathways C 0 …*O 4 , C 0 …O 3 , and C 0 …O 2 after applying fcGMP (red) and after its removal (blue). ( b , c ) Respective pathway net probability fluxes at 2.0 μM and 0.5 μM fcGMP, respectively. Full size image For considering channel deactivation, the opposite pathway net probability fluxes were considered, F p,O2C0 , F p,O3C0 , and F p,*O4C0 (blue arrows in Fig. 6 ). O 2 , O 3 , or *O 4 are now the flux producers and C 0 is the flux collector. O 2 and O 3 can only be emptied along the activation pathway to C 0 because the transition C 3 →C 4 is blocked in the absence of a ligand. In contrast, practically all probability flux collected in *O 4 via the C pathway reaches C 0 along the *O pathway ( Fig. 6a–c ). The consequence is that channel activation and deactivation generated by populating *O 4 is associated with a nearly perfect hysteresis, whereas no hysteresis is associated with the population of O 2 and O 3 . Consequently, maximal liganding and opening of a CNGA2 channel produces an open state *O 4 that basically differs from O 0 ….O 3 . It is clear for long that the function of multimeric allosteric proteins is essentially defined by the cooperative interaction of the subunits. The general understanding of such kind of interaction however is only poor though there has been considerable progress in the past decades in both experimental approaches and computer simulations. Herein, we analysed the function of homotetrameric CNGA2 ion channels in terms of a complex Markovian model and quantified the cooperative interaction of the four equal channel subunits during a complete cycle of activation and deactivation in detail. Methodologically, all tested Markovian models were globally fitted to a set of essentially different data, containing time courses of ligand binding and unbinding as well as channel activation and deactivation, evoked by jumps to three ligand concentrations and back to zero, respectively, in addition to the respective steady-state relationships. It is this manifold of experimental data, and in particular the duality of ligand binding and activation, which was the prerequisite for getting the necessary constraints to identify an appropriate model and to determine a reasonable set of parameters. A similar approach we used previously to specify the subunit action in homotetrameric HCN2 channels pre-activated by a hyperpolarizing voltage [12] . The most important finding of this report is that the fully liganded and activated channel adopts an open conformation *O 4 that qualitatively differs from the open conformations of the partially liganded channel reached during activation (O x ). From *O 4 ligand unbinding along the *O-pathway proceeds ~50 times faster than from the open states O 1 , O 2 , and O 3 along the C-pathway passed after channel closure ( Fig. 3a ). This remarkable result is associated with a pronounced hysteresis for the activation of the fully liganded channel. Because at the saturating concentration of 12 μM fcGMP *O 4 dominates the open states by far ( Fig. 4a , right), this indicates that for high ligand concentrations the hysteresis dominates the activation–deactivation cycle. The reason for the pronounced hysteresis is that during channel activation, starting from C 0 , k C0*O0 is undeterminably slow, leading to a block of the *O-pathway in the forward direction and passage of the C-pathway, whereas during channel deactivation, starting from *O 4 , k *O4C4 is much slower than k *O4*O3 , k *O3*O2 , k *O2*O1 , k *O1*O0 ( Supplementary Table S2 ), leading to a block of the C-pathway and passage of the *O-pathway. Hence, the *O-pathway plays the role of an unbinding bypass. To finally reach C 0 , the slow reaction *O 0 →C 0 has to be passed ( k *O0C0 ). k *O0C0 is similarly slow as k *O4C4 ( Supplementary Table S2 ). Notably, apart from the *O-pathway, essential aspects of the C4L-*O4L model confirm our previous C4L model insofar that only two ligands suffice to fully open the channel ( E 0 , E 1 →0; E 2 , E 3 , E 4 →1) and that the microscopic affinity of the second binding step is critical. Solely these results, but still more the additional *O-pathway, show that the structure and the assumptions of the MWC model [14] , [19] and related models, including the coupled dimer model [20] , are oversimplifying to describe the molecular gating in CNGA2 channels. In the context of ion channel gating, hysteresis was observed previously when an additional slow gating process superimposes with a fast gating process, thereby altering the gating parameters. Theoretically, this can only appear if both processes are coupled. Examples are the voltage gating in alamethicin channels [21] , HERG-channels [22] , NMDA receptors [23] , TRPV3 channels [24] and HCN channels where the phenomenon was termed ‘mode shift’ [25] , [26] . We are not aware that hysteretic gating has been analysed and termed as such in ligand-gated channels. However, the situation is certainly related if activation of the channels is followed by desensitization and if both processes are coupled. In this context, desensitization means that the channel activity decays and that the response of the channel to the ligand conjointly decreases. For the nicotinic receptor desensitization has been studied extensively, thereby showing that desensitization is associated with an increase of the affinity for the ligand [27] , [28] , [29] , [30] , [31] . Furthermore, it has been shown that the recovery rate from desensitization is much faster than desensitization itself. These results led to a cyclic mechanism describing the interplay of activation and desensitization that consists of four states (for review, refer to Sine et al. [32] ). For the ligand gating in HCN2 channels we recently described a complex Markov model with pronounced hysteresis, in which ligand binding proceeds preferentially along the closed states, whereas ligand unbinding proceeds preferentially along the open states, and moreover, activation is facilitated only when one, three or four ligands are bound [13] . The hysteresis observed herein is similarly related to a complex Markov model, the C4L-*O4L model. In contrast to HCN2 channels, the hysteresis identified for the CNGA2 channels employs two types of open states, O x and *O x , of which the *O x states are only reached after the fourth ligand has bound, and for which the binding affinity is essentially reduced. This is also different to the mentioned results in nicotinic receptors, where the complexity of the used models was much lower than in our C4L-*O4L model. We recently demonstrated for the HCN2 channel gating the principle of reciprocity, saying that if ligand binding promotes channel activation then activation promotes ligand binding [17] . We did this by quantifying the affinity increase for fcAMP, a fluorescent ligand analogue to fcGMP, when activating the channels by voltage. However, the principle of reciprocity also means that the ligand binding becomes more tight when the conformational change evoked by the ligand binding has taken place [33] . Hence, in multimeric proteins with multiple binding sites, it is generally assumed that the channel affinity increases in proportion to the number of ligands bound. In HCN2 channels we showed that this is not necessarily the case: The third and fourth ligand are much less tightly bound than the first and the second ligand [12] . Herein we show a more severe derivation from this assumption: In the C4L-*O4L model the affinity depends, of course, on the respective values of K AC but also on the closed–open isomerizations C 2 ↔O 2 and C 3 ↔O 3 that are strongly shifted to the respective open states. Progressive increase of the ligand concentration therefore increases Po because of an increasing recruitment of these closed–open isomerizations. The strong influence of the allosteric transition on the binding affinity has been insightfully demonstrated already for the simple del Castillo–Katz mechanism [33] . Notably, the binding of the fourth ligand evokes opening to an additional open state *O 4 , enabling an additional unbinding pathway, resulting in 50 times faster unbinding ( Fig. 1c ) along the states *O 3 , *O 2 , *O 1 and *O 0 ( Fig. 3a ). This result indicates that completion of the binding by the fourth ligand evokes a wide conformational change in the tetrameric cyclic nucleotide-binding domain (CNBD) affecting all binding sites, possibly by generating a symmetric conformation. Conversely, when the channel is only double or triple liganded, a non-symmetric conformation of the CNBD would lead to a trapping of the ligands by populating O 2 and O 3 . For all these considerations upon hysteresis one should be aware that only during activation with the ligand present, the C4L-*O4L model can reach an equilibrium with a detailed balance, that is, the net flux in the loop of our model is zero. In contrast, after removal of the ligand during deactivation the model is far away from equilibrium and there is no detailed balance. What could be the physiological meaning of a much faster cGMP unbinding from the fully than from the partially liganded open CNGA2 channel? When addressing this question one has to be aware that natural olfactory channels contain two CNGA2 subunits together with one CNGA4 and one CNGB1b subunit and it is a priori not clear whether the CNGA2 subunits work in these natural heterotetrameric channels similarly as in the homotetrameric channels considered herein. When assuming such a similarity, one has to consider that the olfactory channels can be activated by both cAMP and cGMP [2] , [34] . In olfactory sensory neurons it is well established that cAMP essentially contributes to the transmembrane receptor potential by opening CNG channels [35] , [36] , [37] , [38] . However, cGMP is also available and should therefore interfere. cGMP has been reported to participate preferentially in long-term responses [39] , [40] , [41] . The type of cooperation of the two ligands however is still elusive. Concerning our results, one may speculate that the rapid ligand unbinding in the fully activated channel might become relevant for enabling a rapid exchange of the two types of cyclic nucleotides at the fully but not the partially liganded channel. Another speculation is that the described fast ligand unbinding at high ligand concentrations leads to different cellular responses when the cyclic-nucleotide concentrations in the cell change. It seems to be an attractive idea to analyse in future heterotetrameric olfactory channels with a similar approach as used in the present study. Oocyte Preparation and cRNA Injection Oocytes were obtained surgically under anaesthesia (0.3% 3-aminobenzoic acid ethyl ester) from adult females of Xenopus laevis . The procedures had approval from the authorized animal ethical committee of the Friedrich-Schiller University Jena (Germany). The oocytes were treated with collagenase A (3 mg ml −1 , Roche, Grenzach-Wyhlen, Germany) for 105 min in Ca 2+ -free Barth's solution containing (in mM) 82.5 NaCl, 2 KCl, 1 MgCl 2 , 5 HEPES (pH 7.5). After this procedure, oocytes of stage IV and V and were manually dissected and injected with ~50; ng of cRNA encoding WT CNGA2 channels. After injection with cRNA, the oocytes were cultured at 18 °C for 3–4 days in Barth’s solution containing (in mM) 84 NaCl, 1 KCl, 2.4 NaHCO 3 , 0.82 MgSO 4 , 0.41 CaCl 2 , 0.33 Ca(NO 3 ) 2 , 7.5 TRIS, Cefuroxim, Penicillin/Streptomycin (pH 7.4). Confocal patch-clamp fluorometry The fluorescence and the ionic current were measured simultaneously by combining patch-clamp fluorometry [42] with confocal microscopy [10] , [17] . Macroscopic ion currents were recorded with the patch-clamp technique [43] in inside-out patches of Xenopus laevis oocytes expressing bovine homotetrameric CNGA2 channels (accession number: X55010). The patch pipettes were pulled from borosilicate glass tubing with an outer and inner diameter of 2.0 and 1.0 mm (Hilgenberg GmbH, Malsfeld, Germany). The pipette resistance was 0.7–1.2 MΩ. The bath and pipette solution contained (in mM): 150 KCl, 1 EGTA, 5 Hepes (pH 7.4 with KOH). Jumps of the ligand concentration were evoked by a theta-glass pipette mounted on a piezo-driven device [44] generating a laminar flow of a control bath solution and a bath solution including the ligand. The time course of solution exchange at the patch was 5.6±0.6 ms ( n =8; 10–90% rise time; t 10–90 ), as determined from the increase of fluorescence close to the patch membrane when switching from zero to 3 μM fcGMP. This time was in the range of one to two sampling intervals for ligand binding and unbinding and therefore considered to be instantaneous. The duration of the solution pulses was 13.0 s, 7.5 s and 9.0 s at 0.5 μM, 2.0 μM and 12.0 μM fcGMP, respectively. Electrophysiology was controlled by the ISO3 hardware and software (MFK, Niedernhausen, Germany). The sampling rate for current recording was 5,000 Hz and the filter (4-pole Bessel) was set to 2 kHz. The recording voltage was generally set to 10 mV. To monitor the ligand binding, we used 8-DY547-AET-cGMP (fcGMP) as fluorescent ligand [10] , [16] . fcGMP consists of a cGMP to which the fluorescent dye DY547 (Dyomics Jena, Germany) is linked by an aminoethylthio-spacer to position 8 of the guanosine moiety. Recording was performed with the confocal microscope LSM 5 Live (Zeiss, Jena, Germany). The microscope was triggered by the ISO3 software (MFK, Niedernhausen, Germany). The recording rate of the images was 277 Hz. To distinguish in an LSM image the fluorescence of the non-bound fcGMP from that of the bound fcGMP, a second dye, DY647 (ref. 10 ), was added to the bath solution. fcGMP and DY647 were excited with the 532 nm and 635 nm line of a solid-state laser via the AchroGate beam splitter, respectively. The emitted light was split into two channels by a NFT635 dichroic mirror and further filtered by BP550–615 and LP 650 emission filter (Zeiss, Jena, Germany), respectively. The fcGMP molecules bound to the channels in the patch dome were obtained from the fluorescence intensity in the patch dome from which the fluorescence arising from the unbound molecules was subtracted. The procedure has been described previously [10] . This fluorescence, F , was normalized in each patch with respect to the fluorescence F max at the saturating fcGMP concentration of 29.1 μM. Global fit of kinetic models The rate and/or equilibrium constants for a given model were obtained by a global fit to averaged normalized time courses of binding/unbinding and of activation/deactivation, each at 0.5, 2.0 and 12.0 μM fcGMP, as well as to steady-state binding and activation over a wide concentration range. The strategy is described in Supplementary Methods . Statistical analysis Data are given as mean±s.e.m. How to cite this article: Nache, V. et al. Hysteresis of ligand binding in CNGA2 ion channels. Nat. Commun. 4:2866 doi: 10.1038/ncomms3866 (2013).